Bandgap tunability at single-layer molybdenum disulphide grain boundaries Two-dimensional transition metal dichalcogenides have emerged as a new class of semiconductor materials with novel electronic and optical properties of interest to future nanoelectronics technology. Single-layer molybdenum disulphide, which represents a prototype two-dimensional transition metal dichalcogenide, has an electronic bandgap that increases with decreasing layer thickness. Using high-resolution scanning tunnelling microscopy and spectroscopy, we measure the apparent quasiparticle energy gap to be 2.40±0.05 eV for single-layer, 2.10±0.05 eV for bilayer and 1.75±0.05 eV for trilayer molybdenum disulphide, which were directly grown on a graphite substrate by chemical vapour deposition method. More interestingly, we report an unexpected bandgap tunability (as large as 0.85±0.05 eV) with distance from the grain boundary in single-layer molybdenum disulphide, which also depends on the grain misorientation angle. This work opens up new possibilities for flexible electronic and optoelectronic devices with tunable bandgaps that utilize both the control of two-dimensional layer thickness and the grain boundary engineering. Two-dimensional transition metal dichalcogenides (2D TMDs), in particular MX 2 (M=Mo, W; X=S, Se, Te), have attracted much interest recently not only because of their laminar graphene-like packing structure but also their versatile electronic and optical properties. [1] , [2] , [3] , [4] Being atomically thin, they have potential applications for transparent flexible electronics, similar to graphene. However, unlike graphene that does not have a natural bandgap, they offer the possibility of a broad range of semiconducting bandgaps by selecting appropriate 2D binary compounds. Furthermore, 2D TMDs exhibit exotic properties such as indirect-to-direct bandgap crossover with decreasing number of atomic layers [5] , field-induced transport with high on–off ratios [6] , [7] , strong photovoltaic responses [8] , [9] and interesting valleytronics phenomena [10] . Among the most interesting properties of 2D MX 2 materials is the tunability of their electronic structures. For instance, deep gap states can be induced by the presence of defects such as vacancies, lattice antisites, doping and so on [11] , [12] , [13] , [14] . The bandgaps are tunable with layer thickness [15] , [16] , [17] , [18] and stress [19] , [20] , [21] , and edge-dependent semiconducting-to-metallic transitions have been observed [22] , as well as transformations between different stacking geometries [23] , for example, 2H to 1T phase of monolayer molybdenum disulphide (MoS 2 ) [24] . While a small bandgap (few hundred meV) in graphene can be opened by stress and other methods [25] , [26] , the large bandgap tunability of 2D MX 2 materials from a few eV (semiconducting) to 0 (metallic) allow a wide range of applications in a variety of nanoscale and flexible devices. Several studies on atomically thin TMD layers have been performed to characterize their atomic structures and electronic properties. Among them, high-resolution transmission electron microscopy (TEM) is a powerful tool for imaging the crystal lattices [24] , [27] , [28] , [29] , [30] , while photoluminescence (PL) is used to determine the optical bandgap [19] , [20] , [31] , [32] . However, it is the optical exciton or trion states rather than an intrinsic one-electron quasiparticle gap that is being measured in PL spectra. Other experimental tools, including angle-resolved photoemission spectroscopy [15] , [16] and scanning tunnelling microscopy/spectroscopy (STM/STS) [33] , [34] , have been used to probe the intrinsic electronic properties of 2D TMDs. However, due to the stringent requirements of high-quality samples for angle-resolved photoemission spectroscopy and STM/STS measurements, for example, large single-crystalline domains with high uniformity for the former, and clean and atomically flat substrates with adequate conductivity for the later, there has been a lack of high-quality data for the intrinsic electronic properties of MX 2 layers. In this work, the intrinsic electronic properties of MoS 2 atomic layers, especially the bandgap tunability, are studied by high-resolution STM and STS measurements, supported by PL and computational data. The MoS 2 sample was directly grown on a graphite substrate by chemical vapour deposition (CVD) method [27] to avoid contamination introduced by chemical transfer. Large single-crystalline MoS 2 grains with monolayer thickness are formed on the graphite surface. The intrinsic electronic bandgap is determined to be 2.40±0.05 eV for MoS 2 single-layer (SL), which decreases to 2.10±0.05 eV for bilayer (BL) and 1.75±0.05 eV for trilayer (TL). In particular, a novel and unexpected bandgap change with distance with respect to the SL MoS 2 grain boundary (GB) is observed. In contrast to reported TEM GB studies [13] , [30] , where deep gap states were predicted by theoretical calculations, our study shows that the bandgap decreases to 1.55±0.05 eV at the GB with no observable deep gap states when the misorientation angle is 18°. The bandgap increases monotonically away from the GB, reaching that of pristine SL MoS 2 (2.4 eV) at about 4 nm away from the GB. Supported by first-principles calculations, we discuss the underlying mechanism for the changes in bandgap size and band energies in terms of strain effects and charge transfer at the GBs. Atomic and electronic structure of SL, BL and TL MoS 2 The CVD-grown MoS 2 atomically thin film on graphite substrate was degassed overnight at 300 °C in ultra-high vacuum before STM measurements. A typical triangular MoS 2 flake is shown in the large-scale STM image (200 × 200 nm 2 ) in Fig. 1c (refs 27 , 30 , 35 , 36 ). Bare graphite surface is visible everywhere, for example, the lower part of Fig. 1c . A MoS 2 coverage of ~70% is estimated by performing statistical analysis over large areas of the surface. The lateral profile of the MoS 2 flake shown in the inset reveals a height of 7 Å, corresponding to the thickness of one monolayer MoS 2 (ref. 27 ). The edges of the MoS 2 flakes are usually decorated with unknown adsorbates that are difficult to remove even after degassing the sample at higher temperature, that is, 400 °C. This phenomenon is reasonable as the edge sites of MoS 2 are of high chemical reactivity [37] . Fortunately, a clean surface is obtained well within the MoS 2 domain due to its chemical inertness. 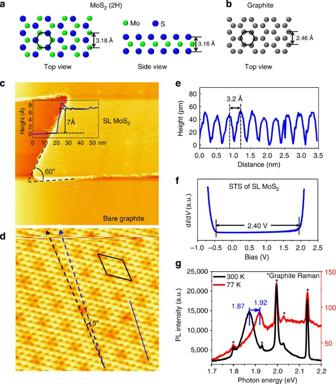Figure 1:Atomic and electronic structure of single-layer MoS2. (aandb) show the atomic structures of monolayer MoS2and graphite, respectively, and their different lattice constants are highlighted. (c) A large-scale STM image (200 × 200 nm2) of a typical triangular single-layer (SL) MoS2island on the graphite substrate (VTip=2.2 V). The inserted lateral profile reveals the height of 7 Å. (d) Moiré superstructure is visible in SL MoS2(8 × 8 nm2;VTip=1.2 V). (e) The lateral profile corresponding to the blue line in panel (d) reveals a 3.2 Å lattice constant of MoS2. (f) STS spectrum reveals a 2.40 eV bandgap for SL MoS2(set point:VTip=1.2 V,ITip=80 pA). (g) PL spectra acquired at 300 K (black) and 77 K (red). The peak for SL MoS2on graphite is located at 1.87 eV at 300 K and shifts to 1.92 eV at 77 K. The other peaks denoted by stars (*) are originating from the graphite substrate. Figure 1: Atomic and electronic structure of single-layer MoS 2 . ( a and b ) show the atomic structures of monolayer MoS 2 and graphite, respectively, and their different lattice constants are highlighted. ( c ) A large-scale STM image (200 × 200 nm 2 ) of a typical triangular single-layer (SL) MoS 2 island on the graphite substrate ( V Tip =2.2 V). The inserted lateral profile reveals the height of 7 Å. ( d ) Moiré superstructure is visible in SL MoS 2 (8 × 8 nm 2 ; V Tip =1.2 V). ( e ) The lateral profile corresponding to the blue line in panel ( d ) reveals a 3.2 Å lattice constant of MoS 2 . ( f ) STS spectrum reveals a 2.40 eV bandgap for SL MoS 2 (set point: V Tip =1.2 V, I Tip =80 pA). ( g ) PL spectra acquired at 300 K (black) and 77 K (red). The peak for SL MoS 2 on graphite is located at 1.87 eV at 300 K and shifts to 1.92 eV at 77 K. The other peaks denoted by stars (*) are originating from the graphite substrate. Full size image Figure 1d shows a high-resolution STM image of SL MoS 2 recorded at a tip bias voltage ( V tip ) of 1.2 V, where a honeycomb structure is demonstrated. A similar honeycomb structure has also been observed for MoSe 2 monolayer on bilayer graphene [34] . The MoS 2 lattice constant of 3.2±0.1 Å is revealed by the line profile in Fig. 1e . The observed Moiré superstructure is attributed to the lattice and/or orientation mismatch between the top-layer MoS 2 and the underlying graphite substrate. As highlighted by the parallelogram in Fig. 1d , the Moiré supercell with dimensions of a = b =12.0±0.4 Å and an intersection angle of 60°±2° approximately corresponds to a (4 × 4) supercell of MoS 2 as well as a (5 × 5) supercell of graphite. The MoS 2 atomic rows are clearly not aligned well with the Moiré pattern, with an angle between both directions of ϕ (MoS2,Moiré) =5°. Many different Moiré patterns coexist in this CVD-grown MoS 2 sample, due to different stacking orientations of the MoS 2 flakes relative to the graphite substrate. Among them, the ϕ (MoS2,Moiré) =5° is the one most frequently observed. The d I /d V spectrum averaged over 100 STS spectra acquired at random points on the SL MoS 2 (far away from the edges and defects) is shown in Fig. 1f . The edge of the valence band maximum (VBM) is located at 1.95±0.03 eV below the Fermi level (FL), and the conduction band minimum (CBM) is located at 0.45±0.03 eV above the FL, thereby yielding an intrinsic one-electron quasiparticle bandgap of E g =2.40±0.05 eV. In contrast, a significantly smaller optical gap is determined from the PL spectra. As shown in Fig. 1g , the PL spectra of the CVD-grown SL MoS 2 on graphite were taken at 300 K (black) and 77 K (red), respectively. The PL peak corresponding to the optical bandgap ( E opt ) of SL MoS 2 is located at 1.87 eV at room temperature and shifts to 1.92 eV at low temperature. The PL peak measured for this CVD sample on graphite is quite close to that reported for SL MoS 2 samples on different substrates [30] , [36] , [38] , indicating that the optical bandgap is relatively insensitive to the nature of the substrate. The other peaks that are marked by star (*) symbols are Raman signals of graphite. An extremely large exciton binding energy, namely the difference between E g and E opt of 0.48 eV is obtained at 77 K (all our STM measurements were performed at this temperature). In a recent study of monolayer MoSe 2 on bilayer graphene, an exciton binding energy as large as 0.55 eV was determined by Ugeda et al [34] . Thus, a strong excitonic binding energy could be a common characteristic for ultrathin 2D MX 2 materials. The substantially reduced dielectric screening of monolayer 2D MX 2 , enhanced Coulomb interactions due to low-dimensional effects and relatively large effective masses of charge carriers there, all contribute to the strong exciton binding energy observed. Furthermore, recent quasiparticle band structure calculations suggested a ~2.9 eV bandgap, and hence a much larger exciton binding energy of ~1.0 eV for free-standing SL MoS 2 (refs 39 , 40 , 41 , 42 ). The difference between our measurements and theoretical calculations is attributed to substrate screening effects, which has also been observed for semiconducting carbon nanotubes on metallic substrates [43] , [44] . The similarity of exciton binding energies obtained for MoS 2 and MoSe 2 both on graphitic substrates might indicate that the metallic substrate plays a dominant role in determining the exciton property for MoX 2 monolayers. Multilayer MoS 2 can also be found in our sample. The large-scale STM image (150 × 150 nm 2 ) in Fig. 2a illustrates a region containing SL, BL and TL MoS 2 , which are highlighted in blue, green and red, respectively. The lateral profile in Fig. 2c reveals a thickness of ~7 Å for each MoS 2 layer. In the atomic-resolved STM image of Fig. 2b , the honeycomb structure of BL MoS 2 is similar to that observed in SL region ( Fig. 1d ). In Fig. 2a , the SL region is obviously composed of many different grains with sizes of between tens of nanometres to a few hundreds of nanometres, and GBs are observed as bright protrusions. These GBs are also visible in the BL and TL regions but with weaker contrast. In contrast to the straight flake edges observed for SL MoS 2 ( Fig. 1c ), the edges of BL and TL islands show curved profiles in Fig. 2a . 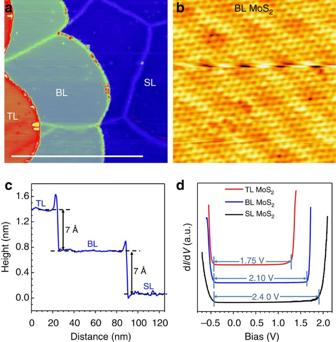Figure 2:Bandgap varying with MoS2layer thickness. (a) Large-scale STM image shows a MoS2flake containing single-layer (SL), bilayer (BL) and trilayer (TL) thickness (150 × 150 nm2;VTip=2.4 V). (b) Highly resolved STM image recorded at the BL region, where the honeycomb feature is similar to that observed for SL MoS2(8 × 8 nm2;VTip=1.5 V). (c) Lateral profile corresponding to the white line in panela, revealing a 7 Å height for each MoS2layer. (d) dI/dVspectra taken at the SL, BL and TL MoS2, respectively, reveals the bandgap decrease with the increasing thickness (set point:VTip=1.5 V,ITip=80 pA). Figure 2: Bandgap varying with MoS 2 layer thickness. ( a ) Large-scale STM image shows a MoS 2 flake containing single-layer (SL), bilayer (BL) and trilayer (TL) thickness (150 × 150 nm 2 ; V Tip =2.4 V). ( b ) Highly resolved STM image recorded at the BL region, where the honeycomb feature is similar to that observed for SL MoS 2 (8 × 8 nm 2 ; V Tip =1.5 V). ( c ) Lateral profile corresponding to the white line in panel a , revealing a 7 Å height for each MoS 2 layer. ( d ) d I /d V spectra taken at the SL, BL and TL MoS 2 , respectively, reveals the bandgap decrease with the increasing thickness (set point: V Tip =1.5 V, I Tip =80 pA). Full size image The edges of the MoS 2 layers usually possess brighter contrast than the terraces, as shown in Fig. 1c (SL) and Fig. 2a (multilayer). The inset of Fig. 1c for SL MoS 2 and Fig. 2c for multilayer films show that peaks with widths of a few nanometres are observable in the lateral profiles at the edges. The bright contrasts recorded at the edges are not artificial, but due to the changes in the local density of states. There are two possible contributions to the changes in the electronic structures at the MoS 2 edges. One is an intrinsic modification of the electronic properties at the edge sites due to the broken periodicity, that is, edge-dependent semiconducting-to-metallic transition for MoS 2 , as predicted by theoretical calculations [22] , [45] . The other contribution is from the guest adsorbates that are often observed at the edge sites due to their higher chemical reactivity. Unfortunately, due to the instability of the MoS 2 edges under STM scanning (due to removal of S atoms), no atomically resolved STM image has been captured so far, so we are unable to determine which mechanism is more likely. STS spectra taken at the SL, BL and TL regions (far away from edges or defects) are shown in Fig. 2d . The bandgap of the MoS 2 film decreases with increasing thickness. The intrinsic 2.40 eV bandgap for SL MoS 2 is reduced to 2.10 eV for BL and further to 1.75 eV for TL. Moreover, it is worth noting that the CBM (left) is pinned at ~0.45 eV above the FL, while the VBM (right) below FL is shifted from 1.95 eV for SL to 1.30 eV for TL. The bandgap decrease with thickness increase of MX 2 is caused by the quantum confinement effect, which has been predicted by density functional theory (DFT) calculations [18] , [39] , and confirmed by optical bandgap measurements [38] . The VBM shifting towards FL with increasing thickness also agrees well with other reported studies of MoS 2 and other 2D TMD materials (for example, MoSe 2 ) using photoemission spectroscopy [15] , [16] . The observed CBM pinning has not been previously reported, and this may have significant implications for device applications of 2D TMD materials. However, the underlying mechanism for this CBM pinning with respect to the MoS 2 thickness is still unclear. Tunable bandgap at SL MoS 2 GB GBs such as that shown in Fig. 2a are critical for 2D TMD materials, as this is where changes of electronic structures are expected. 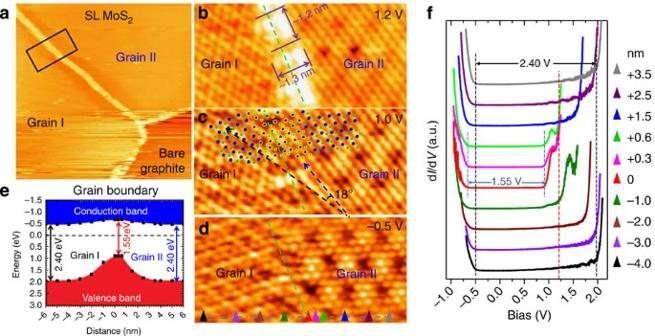Figure 3: Unexpected bandgap tunability at the GB. (a) Large-scale STM image shows a SL MoS2island composed of two grains, where the GB appears as bright protrusions (75 × 75 nm2;VTip=1.5 V).b–dare bias-dependent images recorded at the boundary region highlighted by a black rectangle in panela(8 × 4 nm2;b,VTip=1.2 V;c,VTip=1.0 V;d,VTip=−0.5 V). The misorientation between the grainsIandIIis 18° as determined in panelc. (f) dI/dVspectra recorded at the positions denoted by the triangles in paneld(set point:VTip=1.0 V,ITip=100 pA). The variation of the bandgap with distance from the boundary is quite pronounced. (e) Schematic diagram shows the bandgap change at the GB. Figure 3a shows a typical GB at SL MoS 2 with brighter contrast at V tip =1.5 V. The atomically resolved STM images in Fig. 3b–d clearly reveal different Moiré patterns in grains I and II , that is, ϕ (MoS2,Moiré) of 0° and 5°, respectively. The misorientation between them is 18°±1°, which is similar to that in a reported high-resolution TEM study [13] . The GB is featured as bright protrusions with a width of ~1.3 nm at V tip =1.2 V in Fig. 3b . When V tip is reduced to 1.0 V and −0.5 V in Fig. 3c,d , respectively, the bright features disappear. This suggests that the bright features recorded at higher V tip are not a result of different morphological structure but a change of the electronic states. We observe that the MoS 2 lattice periodicities are discontinuous at the GB and a transition phase possessing different packing structure forms there ( Supplementary Fig. 1 ). As the two grains meet during the CVD process, a possible transition phase of Mo and S, together with other impurities, may form in this 1.3-nm-wide GB region. An atomic structure model proposed in Fig. 3c is overlaid to trace the lattice perturbations (an expanded figure is shown in Supplementary Fig. 2 ). The model suggests that the transition phase between the grains I and II is mainly constructed by distorted MoS 2 lattices. However, as the STM images are convolutions of both surface topology and LDOS information, it is difficult to precisely identify the chemical nature of the transition phase, for example, lattice vacancies/antisites and impurities (such as O) cannot be completely excluded. Figure 3: Unexpected bandgap tunability at the GB. ( a ) Large-scale STM image shows a SL MoS 2 island composed of two grains, where the GB appears as bright protrusions (75 × 75 nm 2 ; V Tip =1.5 V). b – d are bias-dependent images recorded at the boundary region highlighted by a black rectangle in panel a (8 × 4 nm 2 ; b , V Tip =1.2 V; c , V Tip =1.0 V; d , V Tip =−0.5 V). The misorientation between the grains I and II is 18° as determined in panel c . ( f ) d I /d V spectra recorded at the positions denoted by the triangles in panel d (set point: V Tip =1.0 V, I Tip =100 pA). The variation of the bandgap with distance from the boundary is quite pronounced. ( e ) Schematic diagram shows the bandgap change at the GB. Full size image To elucidate the change of the electronic properties, a series of STS spectra were taken across the GB. As displayed in Fig. 3f , the bandgap sizes vary with the distance from the GB, decreasing from the intrinsic 2.40 eV at d ≥4 nm to 1.55 eV at d =0 nm. Here d is defined as the perpendicular distance from the GB regardless of direction (that is, right or left). The middle of the GB, that is, d =0, is denoted by the green dashed lines in Fig. 3b–d . The VBM has a large shift of 1.05 eV towards FL, while the CBM shifts 0.2 eV away from it, resulting in a net change in bandgap of 0.85 eV. As demonstrated in the schematic diagram of Fig. 3e , it is interesting to note that the gap decreases gradually in the range of 2.0< d ≤4 nm, but markedly for 0.6< d <2.0 nm; while for d ≤0.6 nm, the bandgap size is almost constant (1.55 eV) without deep gap states. These observations are consistent with the bias-dependent STM images shown in Fig. 3b–d . For instance, the width of the bright protrusion is found to be ~1.3 nm as denoted in Fig. 3b at V tip =1.2 V and is in good agreement with the fact that d I /d V intensity (proportional to DOS) for d ≤0.6 nm (regardless of direction) is much higher than for d >0.6 nm at V =1.2 V in Fig. 3f (highlighted by a dotted red line). Furthermore, the disappearance of the bright features at the GB in Fig. 3c,d at V tip =1.0 V and −0.5 eV, agrees well with the fact that no pronounced state is detected in this bandgap range and hence no bright feature is observed in the 2D STM contour maps. Another typical GB is shown in Fig. 4 . In the atomically resolved STM image of Fig. 4a , grains III and IV can be distinguished by the orientation difference between the MoS 2 lattices and Moiré patterns, namely ϕ (MoS2,Moiré) , which is denoted by dashed and solid arrows. ϕ (MoS2,Moiré) of grains III and IV are determined to be 20° and 8°, respectively. Careful analysis reveals a very small misorientation of 3° between these two grains. Subsequently, to determine the changes of the electronic properties, STS spectra were measured at the positions marked by the triangles. As shown in Fig. 4b , it is found that similar to the case shown in Fig. 3 , the bandgap E g of 2.40 eV remains constant at d ≥4 nm, and decreases gradually as the tip approaches the GB, for example, 2.23 eV at d =0. The CBMs (left) remain almost constant at −0.45 eV, and the VBMs (right) shift slightly towards to the FL. The bandgap decrease of 0.17 eV observed here is much smaller than that of 0.85 eV for the 18° case shown in Fig. 3 . 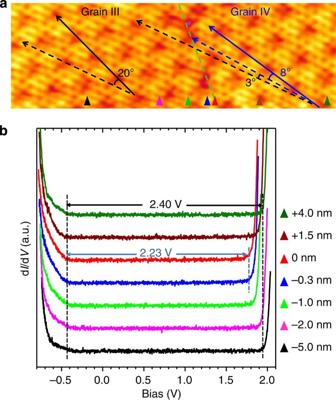Figure 4: Another typical GB with a 3° misorientation. (a) Atomically resolved STM image of grainsIIIandIV. The dashed arrows denote their crystal lattice directions, and the solid arrows denote the Moiré superstructure (12 × 4 nm2;VTip=0.4 V). STS spectra measured at the triangles are shown inb. The bandgap decreases to 2.23 eV at the GB (set point:VTip=−0.8 V,ITip=80 pA). Figure 4: Another typical GB with a 3° misorientation. ( a ) Atomically resolved STM image of grains III and IV . The dashed arrows denote their crystal lattice directions, and the solid arrows denote the Moiré superstructure (12 × 4 nm 2 ; V Tip =0.4 V). STS spectra measured at the triangles are shown in b . The bandgap decreases to 2.23 eV at the GB (set point: V Tip =−0.8 V, I Tip =80 pA). Full size image The fact that no deep gap states are observed in the GB region is in sharp contrast to theoretical predictions [12] . Deep gap states arise because of energetically unfavourable local bonding configurations that are necessary to enable grains of different orientations to come together, that is, non-six-membered rings are suggested to form the line dislocation defects [12] , [30] , [46] . Since no deep gap states are observed, we must conclude that such energetically unfavourable local bonding configurations are not present in the GBs here, indicating that the nature has a better way of healing the defects. One possibility is that adsorbates, such as hydrogen or oxygen, could passivate dangling bonds or satisfy local coordination requirements, moving the defect states closer to the band edges. Furthermore, it is clear that for the large angle mismatch of 18°, the GB region has a fairly wide width of ~1.3 nm, or four lattice constants ( Fig. 3 ), in contrast to previous models with the GB width extending over one lattice constant only. Thus, due to the growth and annealing processes, the GB defects are in fact healed over a much wider region than that considered in simpler models. As discussed below, we believe that this GB defects are accommodated mainly through the lattice distortions that result in a strain field [47] , instead of through energetically unfavourable deep gap states. For the case of 3° GB in Fig. 4 , the MoS 2 lattice orientation changes gradually through the GB without obvious periodicity break and visible defects, suggesting that the strain effect could be the primary reason for the bandgap decrease. As expected, the effects are significantly larger for the GB with 18° misorientation angle than for the GB with 3° misorientation, which is reasonable as a larger mismatch would induce a larger strain field [47] . The STS results indicate that the GB regions have smaller gaps than that of pristine MoS 2 4 nm away from the GBs. A diagram of the bandgap E g versus the distance d away from the GB is plotted in Supplementary Figure 3 . Focusing on the GB with 18° misorientation, we discuss the two possible mechanisms contributing to the decrease of the electronic bandgaps as a function of d . As with previous observations [20] , [41] , [48] , [49] , [50] , [51] , the bandgap of SL MoS 2 is very sensitive to strain, which is thereby first considered here. Line dislocation defects at GBs are well known to be able to create a local strain field [47] , [52] . A recent study on the GBs of monolayer WS 2 suggests that the strain field can extend over several nanometres from the dislocation cores and are at maxima at the dislocation cores where tensile and compressive strains intermix [47] . Since strain is certainly present at and close to the GBs due to the lattice distortions ( Supplementary Figure 2 ), we attribute the change in bandgap with d to strain, the magnitude of which decreases as d increases. In Fig. 5a , we show the change in CBM and VBM energies relative to the vacuum level for free-standing SL MoS 2 as a function of tensile (positive) and compressive (negative) strain, as computed by DFT in the local density approximation (LDA). Although the computed bandgaps are smaller than that determined in experiments (a common error of DFT LDA), we expect the predicted changes in bandgaps to be a good approximation to the corresponding changes in the experimental bandgap, as the self-energy correction to the LDA eigenvalues should be very similar for the same material with moderate amounts of strain. The decrease of the bandgaps, namely the relative changes of the CBM and VBM energies, could be induced by either tensile or compressive strain. While the actual strain field present in experiment is affected by the experimental boundary conditions and interactions with the substrate, we find based on our DFT calculations that the amount of strain required to produce the observed changes in bandgap are reasonably small. Specifically, the estimated strain responsible for the change in bandgap (−0.85 eV) is calculated to be about 4% for biaxial tensile strain, which is well within the range of that described for WS 2 GBs, that is, 5–25% for a 12° GB and 5–58% for a 22° GB [47] . 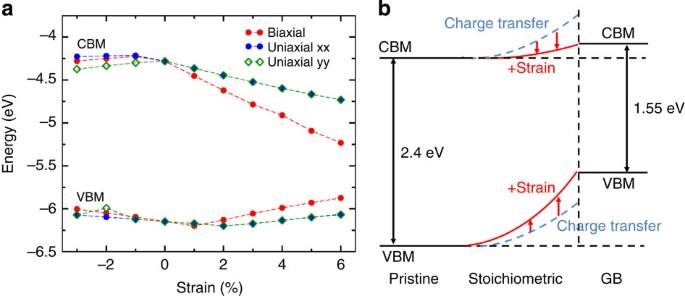Figure 5: A schematic diagram of the bandgap tunability. (a) Strain-induced CBM and VBM changes of pristine monolayer MoS2. The vacuum level is aligned at 0 eV for all strains. (b) Schematic illustration of strain and charge transfer-induced band modulation across the 18° GB. Figure 5: A schematic diagram of the bandgap tunability. ( a ) Strain-induced CBM and VBM changes of pristine monolayer MoS 2 . The vacuum level is aligned at 0 eV for all strains. ( b ) Schematic illustration of strain and charge transfer-induced band modulation across the 18° GB. Full size image We have also considered the possibility of bandgap modulation due to the decay of defect/impurity states from the GB into the interior. A defect may introduce a state near the CBM or VBM, which reduces the bandgap at the GB region, and as the state decays away from the GB, the bandgap widens to the pristine one. The decay behaviour of such a defect state can be predicted by the calculated complex band structure (CBS) of a pristine MoS 2 monolayer (See Supplementary Fig. 4 ). The much smaller decay distance of defect states obtained from the CBS prediction indicates that it is unlikely to be the dominant reason for bandgap modulation there ( Supplementary Note 1 ). Indeed, explicit calculations of different defect states also show that the wavefunctions tend to be localized near the defects [53] , [54] . The long range and smooth nature of the bandgap variation strongly suggest that the strain fields formed around the GBs is the primary contribution to the observed bandgap decrease as a function of distance from the GBs. Furthermore, we note from Fig. 5a that as the bandgap decreases, the electron affinity increases (that is, CBM energy shifts downwards) and ionization energy decreases (that is, VBM shifts upwards), as predicted by theoretical calculations. Since the CBM and VBM are both bending upwards as d decreases, as determined by STS spectra ( Fig. 3e , where FL is located at 0 eV), we can conclude that the changes in CBM and VBM are also influenced by charge transfer effects, either from the substrate [55] or from pristine MoS 2 —a direct consequence of the computed larger electron affinity of strained MoS 2 , to the GB region ( Fig. 5a ). The screening distance of a few nanometres is consistent with previous STS measurements of band bending close to MoS 2 edges [33] . Figure 5b provides a schematic illustration of the above discussion, showing that the unexpected bandgap tunability with distance from the GBs presented here is possibly a result of strain effects combined with defect-/substrate-induced charge transfer. In this high-resolution STM/STS study, we have investigated the intrinsic electronic properties of atomically thin MoS 2 layers directly grown on a graphite surface using CVD method. The electronic bandgap of SL MoS 2 is determined to be 2.40 eV by STS spectra, and hence an extremely large exciton binding energy of 0.48 eV is deduced. The bandgap decreases to 2.10 eV for BL and 1.75 eV for TL MoS 2 , due to quantum confinement effects. Unexpectedly, we find that GBs in SL MoS 2 can heal themselves much better than previously thought during CVD growth, resulting in an absence of deep gap states. Instead, we find that the GB remains semiconducting, and the bandgap and band energies are tunable with respect to the distance to the GB. The decrease of the bandgap at the GB can be as large as 0.85 eV when the misorientation between the two neighbouring grains is 18°, but is only 0.17 eV when the misorientation is 3°. The CBM and VBM also bend upwards from pristine MoS 2 to the GB region, with the effect of band bending increasing for larger misorientation angles. The decreased bandgap and the changes in CBM and VBM energies at the GBs are attributed to a combination of local strain fields, as well as defect-/substrate-induced charge transfer. The unexpected semiconducting nature of MoS 2 GBs, tunable bandgaps and band energies, together with the CBM pinning and large exciton binding energies, provides a more comprehensive understanding of the intrinsic electronic properties of 2D TMD materials. This work allows us to evaluate new possibilities for flexible electronic and optoelectronic devices with tunable bandgaps that utilize both the control of two-dimensional layer thickness and GB engineering. Synthesis MoS 2 crystals were synthesized by a modified CVD process reported previously [27] . In brief, highly oriented pyrolytic graphite substrates were first cleaned by cleaving with 3 M tape before deposition. The substrates were placed in the centre of a 4″ tubular furnace on a quartz holder. MoO 3 (0.6 g; Sigma-Aldrich, 99.5%) precursor in a Al 2 O 3 crucible was placed at 12 cm away from substrates, while S (Sigma-Aldrich, 99.5%) powder in a quartz tube was placed 8 cm away from the furnace open end at an upstream position in a 4″ quartz tube. The furnace was first heated to 150 °C at 10 °C per min rate with 70 s.c.c.m. Ar at 10 torr and annealed for 20 min; the temperature was subsequently increased to 650 °C at 25 °C per min rate and kept for 1 h. Sulphur was heated by a heating belt at 160 °C when furnace reached 400 °C. After growth, the furnace was slowly cooled to room temperature. Characterization STM measurements were carried out in a custom-built multi-chamber ultra-high vacuum system housing an Omicro LT-STM interfaced to a Nanonis controller. The base pressure was better than 10 −10 mbar. A chemically etched tungsten tip was used. The sample was kept at 77 K during all the measurements to obtain better resolution. The STM images were recorded in constant current mode with tunnelling current in the range 50–100 pA. For d I /d V spectra, the tunnelling current was obtained by a lock-in amplifier, with a modulation of 625 Hz and 40 mV. The MoS 2 /graphite sample was degassed at 300 °C overnight before STM analyses. The PL spectra were measured in the back-scattering configuration by a home-made microscopy system. A 532-nm solid-state laser was used as the excitation source, and the laser was focused on the sample by an objective lens with numerical aperture (NA)=0.9 (NA=0.42) for room-temperature (low temperature) measurements. Typically, the laser spot on the sample is ≤1 μm. The PL signals were collected by the same objective lens, analysed by a 0.75-m monochromator and detected by a liquid N 2 cooled CCD camera. For low-temperature PL measurements, the sample was cooled to 10.8 K by a low-vibration cryogen-free cryostat. The sample temperature was controlled by a heater inside the cryostat to 77.0 K with stability of ±0.1 K. Computation First-principles DFT-based methods as implemented in the VASP package [56] were used to investigate the CBM and VBM position dependence of pristine MoS 2 monolayer against tensile and compressive strain. LDA projector-augmented plane-wave pseudopotentials were employed, interatomic forces relaxed to 0.01 eV Å −1 , 16 × 16 × 1 Monkhorst-Pack type k-points sampling was used, plane-wave cutoff energy set at 364 eV and a vacuum space of at least 12 Å was used between the adjacent periodic replications to avoid spurious interaction. The CBS (presented in Supplementary Fig. 4 ) was obtained using the SCARLET code [57] . How to cite this article : Huang, Y. L. et al . Bandgap tunability at single-layer molybdenum disulphide grain boundaries. Nat. Commun. 6:6298 doi: 10.1038/ncomms7298 (2015).